Annexin A2 binds to endosomes following organelle destabilization by particulate wear debris Endosomal functions are contingent on the integrity of the organelle-limiting membrane, whose disruption induces inflammation and cell death. Here we show that phagocytosis of ultrahigh molecular weight polyethylene particles induces damage to the endosomal-limiting membrane and results in the leakage of cathepsins into the cytosol and NLRP3-inflammasome activation. Annexin A2 recruitment to damaged organelles is shown by two-dimensional DIGE protein profiling, endosomal fractionation, confocal analysis of endogenous and annexin A2–GFP transfected cells, and immunogold labelling. Binding experiments, using fluorescent liposomes, confirms annexin A2 recruitment to endosomes containing phagocytosed polyethylene particles. Finally, an increase in cytosolic cathepsins, NLRP3-inflammasome activation, and IL-1 production is seen in dendritic cells from annexin A2-null mice, following exposure to polyethylene particles. Together, the results indicate a functional role of annexin A2 binding to endosomal membranes following organelle destabilization. Late endosomes (LE) and lysosomal compartments are sub-cellular organelles, where functions associated with catabolism of exogenous and endogenous proteins, downregulation of surface receptors, inactivation of pathogenic organisms and loading of processed antigens onto MHC class II molecules take place [1] . All of these specialized functions are contingent on the organelle concentration of numerous hydrolytic enzymes, the presence of an acidic pH, and an organelle-limiting membrane ensuring the anatomical integrity of the compartment [2] . A critical role of the membrane enclosing LE and lysosomes (LYS) is to separate the luminal acid hydrolases from other cellular constituents, thereby protecting them from undesirable degradation. The importance of the integrity of the endosomal/lysosomal organelles is underscored by the severe phenotype associated with the few rare genetic diseases in which the integrity of these compartments is compromised. Among these lysosomal storage diseases are a complex group of pathologies caused by defective metabolic enzymes, which cause aberrant lipid trafficking or catabolism. The overall lipid accumulation impairs endosomal morphology, membrane lipid composition and degradative ability, leading to cell toxicity and death [3] , [4] . Similarly, hyperacidification of endosomes and LYS is observed in cystic fibrosis owing to an efflux of sodium, which increases TLR9 processing, and has been associated with the inflammation observed in this disease [5] . Recently, several studies have demonstrated that endosomal disruption by particulate materials [6] , [7] , [8] , [9] , [10] , or endosomal destabilization by accumulation of aggregates of oxidatively damaged protein/lipids (lipofuscin) [11] , [12] , results in damage of the endosomal-limiting membrane and leakage of cathepsins into the cytosol. A consequence of endosomal disruption by particulates is the assembly and activation of the inflammasome. Inflammasomes are cytosolic macromolecular complexes, which are expressed in inflammatory cells and regulate innate immune responses. Inflammasomes are assembled on recognition of pathogenic challenges, or in response to physically damaging components such as crystalline material. In a series of pathological conditions associated with phagocytosis of particulate debris, such as silicosis, asbestosis, gout and aseptic osteolysis, the phagocytosed particles, (silica, asbestos, uric acid crystals and polyethylene/metal particles, respectively) engorge the endosomal tract and cause physical damage to the endosomal-limiting membrane of mononuclear cells [6] , [7] , [8] , [9] , [10] . Endosomal destabilization results in the leakage of cathepsins into the cytosol, which activates the assembly of the NLRP3 inflammasome either directly or indirectly, through mitochondrial damage and production of reactive oxygen species [13] , [14] . The NLRP3 inflammasome consists of the NLR protein, NLRP3, a cytosolic sensor, which recruits the adaptor molecule ASC that contains a caspase-recruiting domain, and on caspase-1 recruitment, forms the NLRP3 inflammasome complex. The outcome of the complex formation is the caspase-1-dependent processing and secretion of cytokines, including interleukin-1β (IL-1β) and interleukin-18 (IL-18), associated with an overall the induction of an innate inflammatory response [15] . We reasoned that, to avoid an inflammatory response, a cellular repair mechanism could be put in place to seal the endosomal membrane. Wear debris (WD) particles generated at the articulating surface of total joint replacements were employed by our lab to investigate NLPR3 inflammasome activation and endosomal repair mechanisms. We report that phagocytosis of non-biodegradable small WD particles (<10 μm) damage the organelle-limiting membrane with subsequent leakage of endosomal cathepsins into the cytosol and NLRP3 inflammasome activation. Additionally, we present the first evidence that annexin A2 and S100A10 are readily recruited to the endosomal membrane following organelle destabilization. The pivotal role of annexin A2, in promoting this binding, constitutes a cellular attempt to stabilize or reseal the damaged membrane and reduce the NLRP3-mediated inflammatory response. Phagocytosed WD induce NLRP3 inflammasome activation Ultrastructural analysis of periprosthetic tissue recovered from patients undergoing revision surgery indicated that WD particles of different shapes and sizes are present throughout the tissue. The spectrum of particle dimension spanned the nanometre to micrometre size ( Fig. 1a ). Numerous inflammatory infiltrates were also observed in the periprosthetic tissues with phagocytosed nanometre and micrometre size WD particles (arrows) inside their endosomal compartments ( Fig. 1b–d ). WD particles are extremely hydrophobic and have a tendency to embed into lipid membranes [10] , [16] . They persist, even within highly proteolytic micro-environments, as are found within LE and LYS [10] , [11] , [12] , [13] , [14] , [15] , [16] . 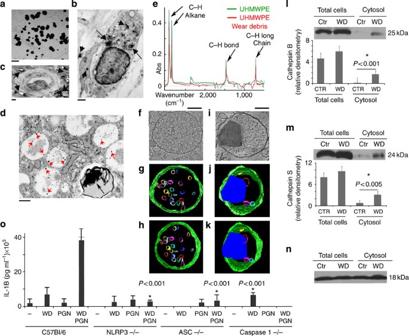Figure 1: NLRP3 inflammasome activation by phagocytosed WD particles. (a) Transmission electron micrograph of nanometre and micrometre size WD recovered from the periprosthetic tissue of patients undergoing joint revision surgery. Bar corresponds to 1 μm. (b) Ultrastructural analysis of micrometre size WD particles (arrows) phagocytosed by myeloid mononuclear cells present in periprosthetic tissue. Bar corresponds to 1 μm. (c) Ultrastructural analysis of micrometre size WD particles (arrows) next to a blood vessel in periprosthetic tissue. Bar corresponds to 1 μm. (d) Ultrastructural analysis of nanometre and micrometre size WD particles (arrows) phagocytosed by a myeloid mononuclear cells present in periprosthetic tissue. Bar corresponds to 500 nm. (e) FTIR spectroscopic analysis of pre-implant UHMWPE and commercially available UHMWPE particles. The analysis was carried out between 4,000 and 500 cm2wave number. (f) Two-dimensional electron micrograph cross-section and (g,h) 3D models derived from 200-nm–section tomograms of an untreated dendritic cell. (g) The late endosome multivesicular body presents a definitive spherical shape and well-defined limiting membrane. (h) The model is rotated 25° relative to (g). (i) 2D electron micrograph cross-section of a micrometre size WD particle phagocytosed by a cultured dendritic cell, and (j,k) 3D tomographic reconstruction of the same (j) WD particle inside the endosomal compartment. (k) The model is rotated 25° relative to (j). (l,m,n) Western blotting for (l) cathepsins B, (m) cathepsin S, and (n) cyclophilin (loading control), from control (Ctr) and WD-particles-treated dendritic cells. Bar graphs represent average and s.e.m. of three independent western blots,P<0.001 andP<0.05 values, respectively, ANOVA, Tukey (o) ELISA for IL-1β secretion from dendritic cells (control, NLRP3, ASC and caspase-1 knockout mice) untreated or treated for 12 h with WD particles (100 μg ml−1), PGN (a TLR2 agonist, at 10 μg ml−1), or WD and PGN combined. The average and s.e.m. of three experiments is shown; asterisk indicates a statistically significant (P<0.001, ANOVA, Tukey) decrease in IL-1 production in NLRP3, ASC and caspase 1 knockout mice as compared with C57Bl/6 controls. Figure 1: NLRP3 inflammasome activation by phagocytosed WD particles. ( a ) Transmission electron micrograph of nanometre and micrometre size WD recovered from the periprosthetic tissue of patients undergoing joint revision surgery. Bar corresponds to 1 μm. ( b ) Ultrastructural analysis of micrometre size WD particles (arrows) phagocytosed by myeloid mononuclear cells present in periprosthetic tissue. Bar corresponds to 1 μm. ( c ) Ultrastructural analysis of micrometre size WD particles (arrows) next to a blood vessel in periprosthetic tissue. Bar corresponds to 1 μm. ( d ) Ultrastructural analysis of nanometre and micrometre size WD particles (arrows) phagocytosed by a myeloid mononuclear cells present in periprosthetic tissue. Bar corresponds to 500 nm. ( e ) FTIR spectroscopic analysis of pre-implant UHMWPE and commercially available UHMWPE particles. The analysis was carried out between 4,000 and 500 cm 2 wave number. ( f ) Two-dimensional electron micrograph cross-section and ( g , h ) 3D models derived from 200-nm–section tomograms of an untreated dendritic cell. ( g ) The late endosome multivesicular body presents a definitive spherical shape and well-defined limiting membrane. ( h ) The model is rotated 25° relative to ( g ). ( i ) 2D electron micrograph cross-section of a micrometre size WD particle phagocytosed by a cultured dendritic cell, and ( j,k ) 3D tomographic reconstruction of the same ( j ) WD particle inside the endosomal compartment. ( k ) The model is rotated 25° relative to ( j ). ( l , m , n ) Western blotting for ( l ) cathepsins B, ( m ) cathepsin S, and ( n ) cyclophilin (loading control), from control (Ctr) and WD-particles-treated dendritic cells. Bar graphs represent average and s.e.m. of three independent western blots, P <0.001 and P <0.05 values, respectively, ANOVA, Tukey ( o ) ELISA for IL-1β secretion from dendritic cells (control, NLRP3, ASC and caspase-1 knockout mice) untreated or treated for 12 h with WD particles (100 μg ml −1 ), PGN (a TLR2 agonist, at 10 μg ml −1 ), or WD and PGN combined. The average and s.e.m. of three experiments is shown; asterisk indicates a statistically significant ( P <0.001, ANOVA, Tukey) decrease in IL-1 production in NLRP3, ASC and caspase 1 knockout mice as compared with C57Bl/6 controls. Full size image To determine whether the phagocytosed debris can damage the endosomal-limiting membrane, we set up in vitro cultures of dendritic cells (DC) exposed to WD particles (0.5–50 μm), whose composition is identical to that of the parent polyethylene compound ( Fig. 1e ). High-resolution electron microscopy and tomographic modelling were employed to examine the endosomal-limiting membrane in contact with the phagocytosed WD particles. In untreated cells, the limiting membrane of endosomal and lysosomal compartments was, as expected, undamaged. A late endosome multivesicular body is shown in Fig. 1f,g , with a classical spherical shape and a well-demarcated limiting membrane, which envelops several luminal vesicles ( Fig. 1f–h ). In contrast, the three-dimensional (3D) analysis of endosomes that have phagocytosed WD particles demonstrated the distortion or distension of the limiting membrane by the phagocytosed particle that appears in part, embedded in the membrane ( Fig. 1i–k ). To determine whether phagocytosis of particulate WD resulted in physical damage to the limiting membrane, the cytosol was isolated from both control and 12-h WD-treated DC, and evaluated by western blotting for the presence of endosomal cathepsins. Western blot analysis detected the presence of cathepsins B and S in the cytosol of WD-treated DC, but not in the cytosol of untreated cells ( Fig. 1l,m ). A known consequence of cathepsin spillage into the cytosol is the activation of the NLRP3 inflammasome. The NLRP3 inflammasome is a multiprotein complex consisted of the NLR protein NLRP3 (a cytosolic sensor), the ASC adaptor, which contains a caspase-recruiting domain, and caspase-1. NLRP3 inflammasome assembly will result in caspase-1 activation, which then processes the immature forms of IL-1β and IL-18 mobilizing them for secretion. Secretion of IL-1β could be detected by ELISA from wild-type C57Bl6 dendritic cells treated with WD particles and peptidoglycan (PGN), but not from the NLRP3 inflammasome component knockout mice (NLRP3, ASC and caspase-1) ( Fig. 1o ). Together, these data indicate that phagocytosed WD can damage the endosomal-limiting membrane with the resultant activation of the NLRP3 inflammasome complex. Annexin A2 recruitment to destabilized endosomes Following WD-induced endosomal destabilization and NLRP3 inflammasome activation, the next experiments were designed to identify proteins involved in endosomal membrane stabilization/repair. two-dimensional (2D)-DIGE protein expression profiling from Cy-dye labelled cytosolic proteins was performed to investigate significant differences in the cytosol from control and WD-treated DC ( Fig. 2a ). As expected, a highly comparable proteomic profile was observed between the two samples; however, a subset of proteins was clearly differentially expressed in the control versus WD-treated cytosol ( Fig. 2b,c ). The most notably downregulated cytosolic protein following WD exposure was annexin A2 ( Table 1 ). Upregulated proteins in the WD-treated sample included proteasomal subunits, and proteases ( Table 1 ). 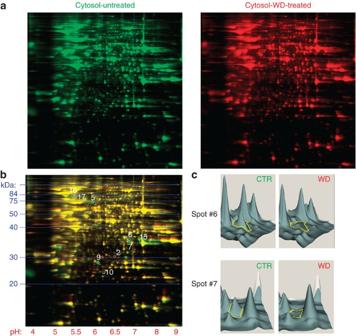Figure 2: Comparative proteomic profiling of cytosol from control and WD-treated DCs. (a) 2D-DIGE protein expression profiling from Cy-dye labelled cytosolic proteins from control and WD-treated DC. (b) An overlay presenting highly comparable proteomic profiles from control and WD-treated cytosol. Circled spots reveal areas of major differences (>threefold) between two samples. (c) 3D-view analysis of protein spots, using 2DCyder software, reveals that the most significantly downregulated cytosolic protein following WD exposure is annexin A2. Figure 2: Comparative proteomic profiling of cytosol from control and WD-treated DCs. ( a ) 2D-DIGE protein expression profiling from Cy-dye labelled cytosolic proteins from control and WD-treated DC. ( b ) An overlay presenting highly comparable proteomic profiles from control and WD-treated cytosol. Circled spots reveal areas of major differences (>threefold) between two samples. ( c ) 3D-view analysis of protein spots, using 2DCyder software, reveals that the most significantly downregulated cytosolic protein following WD exposure is annexin A2. Full size image Table 1 Proteins with >threefold expression difference between the cytosol of untreated or WD-treated DC. Full size table To address the downregulation of annexin A2 from the cytosol of WD-treated DC and examine the possibility of annexin A2 recruitment to the damaged limiting membrane, LE and LYS were isolated from control and WD-treated DC and subjected to western blot analysis ( Supplementary Fig. S1 ). Western blotting demonstrated a substantial increase in annexin A2 presence in the isolated organelles from WD-treated cells as compared with controls ( Fig. 3a,b ). Recruitment of the Ca 2+ binding S100 protein p11 (S100A10) was also observed ( Fig. 3a ). To further confirm annexin A2 recruitment to the endosomal organelles, control and WD exposed DC were stained with LAMP1, as a marker of late endosomal and lysosomal compartments and annexin A2. In control cells, immunofluorescence analysis demonstrated well-defined LAMP1 + endosomal compartments and a cytosolic distribution of annexin A2 ( Fig. 3c ; Supplementary Fig. S2 ). In contrast, WD-treated DC presented enlarged 'doughnut-like' compartments where LAMP1 and annexin A2 completely co-localized ( Fig. 3d ; Supplementary Fig. S2 ). Recruitment of annexin A2 to endosomal compartments containing WD was also observed by ultrastructural analysis following immunogold labelling for annexin A2. In control cells, annexin A2 was mostly evident as a soluble cytosolic protein with some immunogold particles observed in multivesicular late endosomes ( Fig. 3e ). On the other hand, increased recruitment of endosomal annexin A2 was observed around compartments containing phagocytosed particles ( Fig. 3f,g ). To further confirm these results, DC were transfected with annexin A2–GFP complementary DNA. Two days following transfection, DC were exposed to WD for 12 h, or left untreated, and stained for the endosomal marker LysoTracker ( Fig. 3h,i ). In control cells, annexin A2–GFP was mostly observed in the cytosol ( Fig. 3h , Supplementary Fig. S3 ). In contrast in WD-treated DC, LysoTracker and annexin A2 almost completely co-localized ( Fig. 3i ; Supplementary Fig. S3 ). Time-lapse microscopy was also performed on annexin A2–GFP transfectants following phagocytosis of WD particles. In these experiments, we focused on cells where WD particles of at least 0.5–1 μm could be observed on the cell surface at the beginning of the experiments. Debris particles of diameter of around 0.5–1 μm could still be visualized, because they are highly birefringent. Their presence on the cell surface at time 0 helped to predict which cells were likely to phagocytose the WD particles. Twenty-to-forty minutes following phagocytosis of particles, we observed great enlargement of LysoTracker-positive compartments with loss of crisp image morphology. Cellular diffusion of the LysoTracker, with concomitant recruitment of annexin A2 to the site then ensued in the most cells observed ( Fig. 3j,k; Supplementary Fig. S4 ). Together, these results indicate that endosomal compartments disrupted by phagocytosed WD particles recruit cytosolic annexin A2. 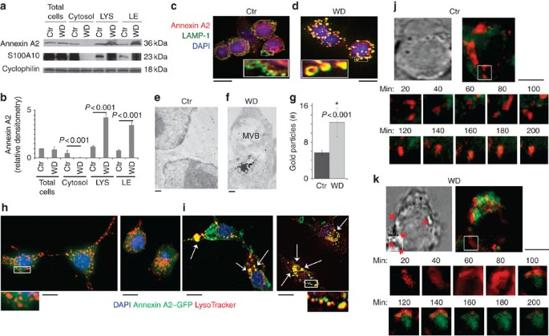Figure 3: Phagocytosis of WD particles results in Annexin A2 recruitment to LE and Lys. (a) Western blot analysis of annexin A2 and S100A10 localization in LE and LYS isolated from WD-treated DCs. (b) Bar graphs represent average and s.e.m. (P<0.001, ANOVA Tukey) of densitometric analysis of three independent western blots. (c,d) Confocal analysis of (c) untreated and (d) 12 h WD-treated DC stained with anti-LAMP1 (green) and anti-annexin A2 (red) revealed well-delineated LAMP+endosomal compartments with cytosolic distribution of annexin A2 in control cells. DC cultured with WD, for 12 h, demonstrated an extensive increase in the number and size of the endosomal compartments with the subsequent loss of the cytosolic distribution of annexin A2. Bar corresponds to 10 μm. (e,f) Ultrastructural analysis of DC immunogold labelled with annexin A2 mAb. (e) In CTR cells, annexin A2 is mostly cytosolic. Bar corresponds to 500 nm. (f) In DC with phagocytosed WD, several annexin A2 gold particles are observed around the compartments with internalized WD particles. Bar corresponds to 200 nm. (g) Quantification of the annexin A2 immunogold labelling observed on the limiting membrane of endosomal compartments in Ctr and WD-treated cells (Values are mean+s.e.m. of three different experiments with >30 cells counted per experiment.P<0.001, ANOVA-Tukey). (h,i)Fluorescent microscopic analysis of annexin A2–GFP-transfected DCs stained with LysoTracker (red) (h) revealed well-delineated endosomal compartments with cytosolic distribution of annexin A2 in control cells. (i) DC cultured with WD, for 12 h, demonstrated an extensive increase in the size of the endosomal compartments with co-localization between LysoTracker and annexin A2. Bars corresponds to 10 μm. (j,k) Time-lapse microscopy of control and 12-h WD-treated DC. (j) Control cells demonstrated a mostly non-overlapping distribution of annexin A2–GFP and LysoTracker. (k) In WD-treated cells, endosomal destabilization and LysoTracker leakage is observed at around 40–60 min, followed by annexin A2 endosomal recruitment lasting up to 200 min. Bars corresponds to 10 μm. Figure 3: Phagocytosis of WD particles results in Annexin A2 recruitment to LE and Lys. ( a ) Western blot analysis of annexin A2 and S100A10 localization in LE and LYS isolated from WD-treated DCs. ( b ) Bar graphs represent average and s.e.m. ( P <0.001, ANOVA Tukey) of densitometric analysis of three independent western blots. ( c , d ) Confocal analysis of ( c ) untreated and ( d ) 12 h WD-treated DC stained with anti-LAMP1 (green) and anti-annexin A2 (red) revealed well-delineated LAMP + endosomal compartments with cytosolic distribution of annexin A2 in control cells. DC cultured with WD, for 12 h, demonstrated an extensive increase in the number and size of the endosomal compartments with the subsequent loss of the cytosolic distribution of annexin A2. Bar corresponds to 10 μm. ( e , f ) Ultrastructural analysis of DC immunogold labelled with annexin A2 mAb. ( e ) In CTR cells, annexin A2 is mostly cytosolic. Bar corresponds to 500 nm. ( f ) In DC with phagocytosed WD, several annexin A2 gold particles are observed around the compartments with internalized WD particles. Bar corresponds to 200 nm. ( g ) Quantification of the annexin A2 immunogold labelling observed on the limiting membrane of endosomal compartments in Ctr and WD-treated cells (Values are mean+s.e.m. of three different experiments with >30 cells counted per experiment. P <0.001, ANOVA-Tukey). ( h , i) Fluorescent microscopic analysis of annexin A2–GFP-transfected DCs stained with LysoTracker (red) ( h ) revealed well-delineated endosomal compartments with cytosolic distribution of annexin A2 in control cells. ( i ) DC cultured with WD, for 12 h, demonstrated an extensive increase in the size of the endosomal compartments with co-localization between LysoTracker and annexin A2. Bars corresponds to 10 μm. ( j , k ) Time-lapse microscopy of control and 12-h WD-treated DC. ( j ) Control cells demonstrated a mostly non-overlapping distribution of annexin A2–GFP and LysoTracker. ( k ) In WD-treated cells, endosomal destabilization and LysoTracker leakage is observed at around 40–60 min, followed by annexin A2 endosomal recruitment lasting up to 200 min. Bars corresponds to 10 μm. Full size image Annexin A2-liposome binding to destabilized endosomes To quantify the effects of the presence of WD on annexin A2 recruitment to endosomal compartments, an in vitro binding assay was set up between gradient-purified late endosomes ( Supplementary Fig. S1 ) derived from untreated or WD-treated DC, and fluorescent liposomes of defined composition assembled in the presence or absence of annexin A2. Typical endosomal compartments visualized by fluorescence-activated cell sorting (FACS) analysis before or after binding with fluorescent liposomes are depicted in Fig. 4a,b . Liposomes were prepared using either phosphatidylserine (PS) or PS and cholesterol, because both lipids are well-known annexin A2 binders. Liposomes were also prepared in the absence or presence of annexin A2. PS and PS/cholesterol liposome binding to endosomes was negligible ( Fig. 4c,d ). In both liposomal preparations, the presence of annexin A2 greatly increased the extent of liposome–endosome binding ( Fig. 4c,d ). The binding was further increased in endosomes prepared from cells that had previously phagocytosed WD ( Fig. 4c,d ). 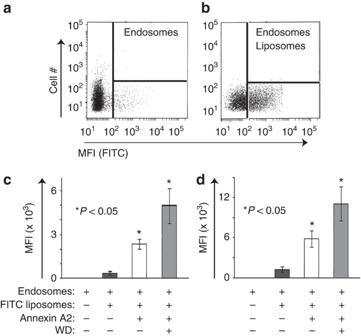Figure 4: Endosomal WD increase fusion between endosomes and annexin A2 liposomes. (a) FACS analysis of purified endosomal compartments. (b) Representative FACS analysis of endosomal compartments following incubation with FITC-liposomes. (c) Mean fluorescence index of endosomes incubated with PS-FITC liposomes in presence or absence of annexin A2 and WD. The graph represents the mean and s.d. of three independent experiments (P<0.05, ANOVA, Tukey). (d) Mean fluorescence index of endosomes incubated with PS/Chl-FITC liposomes in the presence or absence of annexin A2 and WD particles. The graph represents the average of three independent experiments. Asterisks indicate a statistically significant increase in endosomal–liposomal fusion in each of the reported experimental conditions.P<0.05, ANOVA, Tukey. Figure 4: Endosomal WD increase fusion between endosomes and annexin A2 liposomes. ( a ) FACS analysis of purified endosomal compartments. ( b ) Representative FACS analysis of endosomal compartments following incubation with FITC-liposomes. ( c ) Mean fluorescence index of endosomes incubated with PS-FITC liposomes in presence or absence of annexin A2 and WD. The graph represents the mean and s.d. of three independent experiments ( P <0.05, ANOVA, Tukey). ( d ) Mean fluorescence index of endosomes incubated with PS/Chl-FITC liposomes in the presence or absence of annexin A2 and WD particles. The graph represents the average of three independent experiments. Asterisks indicate a statistically significant increase in endosomal–liposomal fusion in each of the reported experimental conditions. P <0.05, ANOVA, Tukey. Full size image Acidification and Ca 2+ release following endosomal destabilization The confirmation of annexin A2 recruitment to the endosomes of WD-treated DC led to the next series of experiments aimed at addressing the mechanism(s) underlying annexin A2 binding to the organelle-limiting membranes. Annexin A2 binds acid phospholipids (among which PS is the best characterized) in a Ca 2+ -dependent manner. On the other hand, annexin A2 cholesterol binding has been shown to be Ca 2+ independent [17] . Recent reports indicate that H + ions may also favour annexin A2 binding to membrane lipids [18] , [19] . To determine possible changes in pH and Ca 2+ in the cytosol of WD-treated cells, direct microelectrode measurements and spectrofluorometric assays, with a pH-sensitive lysosensor probe, were performed. Lysosensor dye (which becomes more fluorescent in acidic environments) indicated a reduction in the cytosolic pH of DC treated with WD for 12 h ( Fig. 5a ). A decrease in pH was also observed by direct pH measurement, using microelectrodes ( Fig. 5b ). Likewise, Ca 2+ measurements revealed a tenfold increase in the cytosolic calcium levels in the WD-treatment group compared with the control ( Fig. 5c ). To analyse lipid binding by annexin A2, a variety of liposomes were prepared that included phosphatidylcholine, a lipid known to be a non-annexin A2 binder, PS, and PS:cholesterol (PS Chl), both of which are well-characterized annexin A2 binders ( Fig. 5d ). Ellipsometry tracings of annexin A2 at physiological pH illustrated that binding to PS and PS-Chl bilayers is greatly enhanced by calcium. In the absence of Ca 2+ , some annexin A2 binding was observed with PS-Chl liposomes but not in the PS liposomes ( Fig. 5e ). At slightly acidic pH (pH 7.15), ellipsometry studies indicate a pH-dependent effect on annexin A2 binding to PS-Chl liposomes, which occurred even in the absence of Ca 2+ ( Fig. 5f ). An additive effect of lower pH and higher calcium on annexin A2 binding to PS and PS-Chl liposomes was observed, as the combination of calcium and pH elicited the strongest binding of annexin A2 to PS-Chl liposomes followed by PS ( Fig. 5f ). In a second approach, western blot analysis was performed on defined liposomes that were incubated with annexin A2 in the presence or absence of Ca 2+ at different pH values, and subsequently pelleted by ultracentrifugation. Western blot determinations of bound and unbound annexin A2 confirmed the findings from the ellipsometry studies under all conditions tested ( Fig. 5g,h ). 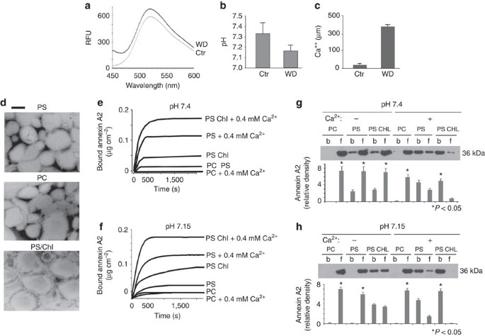Figure 5: WD exposure reduces pH and increases Ca++levels in cytosol of DC. (a) Lysosensor green fluorescent pH measurement of cytosol isolated from control and WD-treated cells (one out of three experiments is shown). (b) Microelectrode pH measurement of media from control and WD particle-treated cells. (mean+s.e.m. were calculated from five different experiments.,P<0.05, ANOVA, Tukey) (c) Calcium measurement in the cytosol from control and WD particle-treated cells. (mean+s.e.m. were calculated from three different experiments.,P<0.001, ANOVA, Tukey) (d) Electron micrograph of negative staining of various liposomes prepared for ellipsometry studies. Bar corresponds to 100 nm. (e,f) Ellipsometry tracings of annexin A2 binding to liposomes under a variety of conditions. (e) Ellipsometry tracing shows annexin A2 (5 μg ml−1) binding to various phospholipid bilayers at physiological pH in the presence or absence of Ca++, (1 out of 4 different experiments is shown). (f) ellipsometry tracing displays annexin A2 (5 μg ml−1) binding to various phospholipid and cholesterol bilayers at acidic pH in presence or absence of Ca++(1 out of 4 different experiments is shown). (g,h) Western blot analysis, with related densitometric analysis, of liposomes incubated with annexin A2 in the presence or absence of Ca++and at different pH values, and subsequently pelleted by ultracentrifugation (b=bound and f=free or unbound annexin A2), (mean+s.e.m. were calculated from 4 different experiments.,P<0.05, ANOVA, Tukey). Figure 5: WD exposure reduces pH and increases Ca ++ levels in cytosol of DC. ( a ) Lysosensor green fluorescent pH measurement of cytosol isolated from control and WD-treated cells (one out of three experiments is shown). ( b ) Microelectrode pH measurement of media from control and WD particle-treated cells. (mean+s.e.m. were calculated from five different experiments., P <0.05, ANOVA, Tukey) ( c ) Calcium measurement in the cytosol from control and WD particle-treated cells. (mean+s.e.m. were calculated from three different experiments., P <0.001, ANOVA, Tukey) ( d ) Electron micrograph of negative staining of various liposomes prepared for ellipsometry studies. Bar corresponds to 100 nm. ( e , f ) Ellipsometry tracings of annexin A2 binding to liposomes under a variety of conditions. ( e ) Ellipsometry tracing shows annexin A2 (5 μg ml −1 ) binding to various phospholipid bilayers at physiological pH in the presence or absence of Ca ++ , (1 out of 4 different experiments is shown). ( f ) ellipsometry tracing displays annexin A2 (5 μg ml −1 ) binding to various phospholipid and cholesterol bilayers at acidic pH in presence or absence of Ca ++ (1 out of 4 different experiments is shown). ( g , h ) Western blot analysis, with related densitometric analysis, of liposomes incubated with annexin A2 in the presence or absence of Ca ++ and at different pH values, and subsequently pelleted by ultracentrifugation (b=bound and f=free or unbound annexin A2), (mean+s.e.m. were calculated from 4 different experiments., P <0.05, ANOVA, Tukey). Full size image Increased NLRP3 inflammasome activation in annexin A2-null mice Finally, we wished to determine whether the absence of annexin A2 would further compromise endosomal integrity following phagocytosis of WD particles. To this end, DC were prepared from annexin A2-null mice and wild-type controls ( Fig. 6a–d ). Cells were left untreated or incubated with WD particles for 12 h. Endosomal damage was quantified as cathepsin B leakage as well as IL-1 production, both of which are indicators of inflammasome activation. Cathepsin B release increased by 30–40% in cells from annexin A2-null mice, as compared with control cells ( Fig. 6e,f ). Similarly, a statistically significant increase in IL-1 production was observed in annexin A2-deficient WD-exposed cells as compared with controls ( Fig. 6g ).Together, these data support the functional relevance of annexin A2 in counteracting endosomal damage, or increase endosomal stabilization following exposure to WD ( Fig. 7 ). 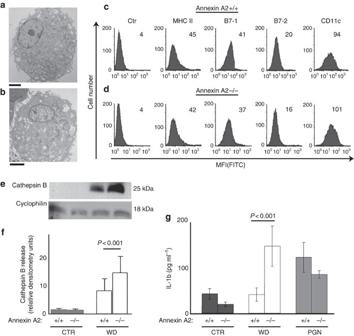Figure 6: Increased inflammasome activation in annexin A2 knock out mice. (a) Ultrasctructural analysis of annexin A2+/+ DC. Bar correspond to 2 μm. (b) Ultrasctructural analysis of annexin A2−/− DC. Bar correspond to 2 μm. (c) FACS analysis of DC surface markers on annexin A2+/+ DC. (d) FACS analysis of DC surface markers on annexin A2−/− DC. (e) Western blot analysis and (f) densitometry analysis of cytosolic cathepsin B in control CTR and WD-treated DC. The mean and s.e.m. of three experiments is shown (P<0.001, ANOVA, Tukey). (g) ELISA for IL-1β secretion from untreated and WD-treated DC (12 h), and from wild type DC and DC deficient in PGN (a TLR2 agonist). The mean and s.e.m. of four experiments is shown (P<0.001, ANOVA, Tukey). Figure 6: Increased inflammasome activation in annexin A2 knock out mice. ( a ) Ultrasctructural analysis of annexin A2+/+ DC. Bar correspond to 2 μm. ( b ) Ultrasctructural analysis of annexin A2−/− DC. Bar correspond to 2 μm. ( c ) FACS analysis of DC surface markers on annexin A2+/+ DC. ( d ) FACS analysis of DC surface markers on annexin A2−/− DC. ( e ) Western blot analysis and ( f ) densitometry analysis of cytosolic cathepsin B in control CTR and WD-treated DC. The mean and s.e.m. of three experiments is shown ( P <0.001, ANOVA, Tukey). ( g ) ELISA for IL-1β secretion from untreated and WD-treated DC (12 h), and from wild type DC and DC deficient in PGN (a TLR2 agonist). The mean and s.e.m. of four experiments is shown ( P <0.001, ANOVA, Tukey). 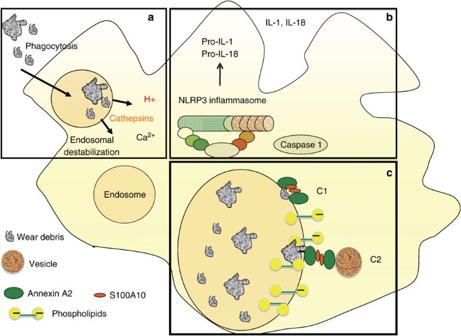Figure 7: Model of annexin A2 binding to endosomes. (a) Phagocytosed WD induce endosomal damage and leakage of cathepsins, Ca++and H+into the cytosol. (b)Endosomal destabilization induces activation of NLRP3 inflammasome, which activates caspase 1 to cleave pro IL-1 and pro IL-18 into mature, secreted IL-1 and IL-18 (c) Cytosolic annexin A2 and S100A10 are recruited to the endosomal membrane as an attempt to restore membrane integrity. C1: The (annexin A2-S100A10)2complex bridges submicrometre membrane gaps. C2: The (annexin A2-S100A10)2complex recruits cytosolic vesicles to bridge micrometre size gaps. Full size image Figure 7: Model of annexin A2 binding to endosomes. ( a ) Phagocytosed WD induce endosomal damage and leakage of cathepsins, Ca ++ and H + into the cytosol. ( b) Endosomal destabilization induces activation of NLRP3 inflammasome, which activates caspase 1 to cleave pro IL-1 and pro IL-18 into mature, secreted IL-1 and IL-18 ( c ) Cytosolic annexin A2 and S100A10 are recruited to the endosomal membrane as an attempt to restore membrane integrity. C1: The (annexin A2-S100A10) 2 complex bridges submicrometre membrane gaps. C2: The (annexin A2-S100A10) 2 complex recruits cytosolic vesicles to bridge micrometre size gaps. Full size image Previously, we reported a model of endosomal disruption following phagocytosis of WD particles, generated by the wear and tear of joint replacement devices [10] , [16] . In this study, high-resolution electron microscopy and tomographic modelling revealed that phagocytosed WD induced distortion and damage of the organelle's limiting membrane, with subsequent leakage of endosomal cathepsins in the cytosol. This results in direct or indirect (via mitochondrial damage and production of reactive oxygen species) assembly and activation of the NLRP3 inflammasome complex [13] , [14] . To investigate proteins recruited to the damaged organelle-limiting membrane, 2D-DIGE protein expression profiling was performed using Cy-dye labelled cytosolic proteins from control and WD-treated cells. Within the cytoplasm, annexin A2 was found to be the most downregulated protein following exposure to WD particles. Fluorescence microscopy and western blot analysis confirmed the extensive recruitment of annexin A2 to the organelles' limiting membrane. The annexins are a family of structurally analogous proteins found in all eukaryotes. Annexins are characterized by their ability to bind acidic phospholipids in a Ca 2+ -dependent manner, and by their prominent alpha helical protein core [20] , [21] . The Ca 2+ -binding sites, located in the carboxy-terminus, are highly conserved among all annexins, and comprise a core, shaped as a slightly curved disk, which contains few Ca 2+ and lipid-binding domains accessible for membrane binding. In contrast, the amino-terminal domain is heterogeneous and endows each annexin with its unique function [22] , [23] . Recently, a series of studies on plasma membrane damage have indicated that annexin A1 and A2 mediate repair mechanisms. Both annexin A1 and annexin A2 have been shown to interact with dysferlin in promoting skeletal muscle sarcolemmal wound repair [24] . Annexin A2 surface translocation has been observed in mechanically damaged human epithelial airway cells [25] , and alveolar type II cells exhibited a decrease in membrane fusion activity when cytosolic annexin A2 was depleted [26] . Annexin A1 has also been shown to be required for the plasmalemmal repair of HeLa cells subjected to laser-induced disruption, and to repair damaged intestinal mucosa [27] . Similarly, cells expressing mutant annexin A1, incapable of binding Ca 2+ , failed to reseal the membrane disruption [28] . Herein, we demonstrate that annexin A2 is also recruited during endosomal destabilization following phagocytosis of particulate material. Annexin recruitment to the organelle-limiting membrane could be important in stabilizing the endosomal membrane and/or containing proteolytically active cathepsins within the organelles. The well-characterized model of annexin A2 binding to a single membrane, which requires only the core domain, containing Ca 2+ /PS binding sites, cannot explain the bridging between two separate membranes, as required during membrane repair. To explain annexin A2-mediated membrane bridging, it has been postulated that, in the presence of Ca 2+ and at pH 7.4, the conserved Ca 2+ -binding domains, within the core domain of an annexin A2 dimer [19] , [29] , [30] , mediate electrostatic interactions with PS located in the membrane to be fused, whereas the Ca 2+ -binding S100A10 stabilizes the annexin A2 dimer, thus bridging the gap between the two membranes [19] ( Fig. 7c ). Indeed, in vitro experiments have shown that formation of the heterotetrameric complex (annexin A2-S100A10) 2 is sufficient to aggregate membranes [31] . However, when membrane disruption is in the micrometre range, the A2-S100A10 heterotetramer cannot bridge the membrane gap. Under such circumstances, it is likely that (A2-S100A10) 2 mediates a stabilization/repair mechanism that involves homotypic vesicle fusion from the cytosol [32] , [33] . ( Fig. 7c ). Through an exocytotic mechanism, these patch vesicles would anneal to the disruption site, establishing barrier continuity [31] ( Fig. 7c ). In both cases, promoting fusion between an incoming vesicle and the disrupted membrane, or closing a gap between two membranes, requires the presence of two lipid-binding sites [19] , [28] , [34] . Recently, several reports have indicated that, at least in vitro , (A2-S100A10) 2 can bind lipid membranes independently of Ca 2+ ions, but in the presence of H + (refs 18 , 35 , 36 , 37 ). Our model supports this hypothesis because, in endosomal organelles disrupted by WD phagocytosis, increased annexin A2 endosomal binding is also associated with increased S100A10 recruitment. As with the pH changes observed during intracellular hypoxia [38] , endosomal disruption generates a locally acidic micro-environment that favours annexin A2-S100A10-mediated membrane aggregation [38] . Finally, Ca 2+ - and H + -independent, but cholesterol-dependent, annexin A2 endosomal binding has also been suggested [39] . Our results demonstrating annexin A2 binding to PS/Chl liposomes support this notion. Even though, based on our experimental data, we hypothesize that annexin A2-Chl binding has a major role during endosomal trafficking, at physiological conditions (low Ca 2+ and normal pH) than during events of membrane disruption (high Ca 2+ and acidic pH. In conclusion, our analysis is the first to establish in a cellular setting that annexin A2 can bind damaged endosomal membrane in a Ca 2+ - and/or H + -dependent manner. More importantly, the data reveal that, following membrane damage due to internalization of WD particles, annexin A2 participates in endosomal membrane stabilization or repair, thereby curtailing inflammasome activation and IL-1 production. These data suggest a role for annexin A2 in modulating the innate inflammatory response. Mice and DC preparation Bone marrow was collected from the femurs of C57BL6, NLRP3−/−, ASC−/− , Caspase-1−/− and Annexin A2−/− mice. Animal euthanasia and organ collecting were carried out according to a protocol approved by the Institutional Animal Care of Albert Einstein College of Medicine. Bone marrow cells were differentiated in GM-CSF (10 ng ml −1 , RD Systems) for 8 days. Preparation of WD WD particles ( Fig. 1a ) were purified from the periprosthetic tissue by sonication and papain digestion at 64 °C for 72 h, followed by serial centrifugation, filtration and ethanol washes [16] . Ultrahigh molecular weight polyethylene was acquired from Sigma-Aldrich (cat #434272) [10] . Fourier transform infra-red spectroscopic analysis Pre-implant ultrahigh molecular weight polyethylene (UHMWPE) and commercially available UHMWPE (Sigma) were analysed by Fourier transformed infrared (FTIR) spectroscopy using a JASCO 6100 Infrared Spectrometer equipped with a Golden Gate attenuated total reflectance cell [16] . Transmission electron microscopy and electron tomography Periprosthetic tissue was fixed in 2.5% glutaraldehyde, 2% paraformaldehyde, in sodium cacodylate buffer 0.1 M, pH 7.4 for 3 h at 4 °C and embedded in LX112-Araldite (Ted Pella Inc, CA, USA). Ultrathin sections were stained with uranyl acetate followed by lead citrate, and viewed with a Jeol JEM-1200EX transmission electron microscope (Jeol Ltd., Akishima, Japan) at 80 kV. Tomographic analysis was performed on 200 nanometre thick sections labelled with 15 nanometre fiducial gold applied to both sides of the sections for alignment of the tilt series. Tomograms were imaged on a Tecnai 20 FEI at ×7,800. Contouring models of the limiting membrane and vesicles were generated through IMOD-guided tracking of prominent contrasted lines and planes in the tomograms [17] . Immunogold labelling DC, untreated or exposed to WD for 12 h, were fixed in 3.7%. paraformaldehyde, 0.1% glutaraldehyde in dPBS, permeabilized in 0.1% Triton-X-100 and blocked in 1% FBS, 1% BSA in dPBS (blocking buffer). Cells were then incubated overnight with 4 μg ml −1 of goat anti mouse annexin A2 antibody (clone A-15, Santa Cruz Biotechnology), followed by 0.8 μg ml −1 of ultrasmall gold-conjugated rabbit anti goat IgG (Electron Microscopy Sciences, Hatfield, PA). Ultrasmall gold conjugates were enhanced with the Aurion R-Gent SE-EM kit (Electron Microscopy Sciences). Samples were viewed with a Jeol JEM-1200EX transmission electron microscope (Jeol) at 80 kV. Organelles fractionation and cytosol preparation LE and LYS were purified using a 10, 27% two-step sucrose gradient [17] . Cytosol was prepared from homogenates following centrifugation for 1 h at 100,000 g . Western blot analysis Cells were lysed in 150 mM NaCl, 50 mM Tris, 1 mM EDTA and 1% NP40. Lysates were run on 12% SDS–PAGE and transferred membranes were incubated with the following antibodies: anti cathepsin B (1 μg ml −1 , clone S-12), anti cathepsin S (1 μg ml −1 , clone C-19), anti annexin A2 (1 μg ml −1 , clone A-15) anti S100A10 (1 μg ml −1 , clone N-16) anti cyclophilin (1 μg ml −1 , clone C14) all from Santa Cruz. Secondary antibody was bovine anti-goat IgG-HRP (0.1 μg ml −1 ) (Santa Cruz Biotechnology). Membranes were developed using chemiluminescent kit (Pierce). Production of recombinant annexin A2 Annexin A2 cDNA was amplified by RT–PCR using the following primers: forward: AGCGGATCC ATGTCTACTGTCCACG (bases from 75 to 90 on annexin A2 messenger RNA) and reverse: AGCCTGCAGTCAGTCATCCCCACC (bases from 1079 to 1094 on annexin A2 mRNA) Following confirmatory sequencing, generated clones were inserted in the BamHI and PstI sites of pTrcHis A vector (Invitrogen) for the production of recombinant proteins. Recombinant annexin A2 was purified by fast protein liquid chromatography. Dendritic cell transfection with annexin A2–GFP Annexin A2–GFP cDNA was purchased from OriGene (OriGene Technologies, Catalogue No MG205064). DC cultured in DMEM medium, supplemented with 10% FBS, were transfected with the cDNA (4 μg plasmid DNA/ 2×10 6 cells) encoding annexin A2–GFP fusion protein using Lipofectamine 2000 (Invitrogen). Immunofluorescence and Time-lapse fluorescence microscopic analysis DCs were either left untreated or exposed to WD for 12 h. Cells were then fixed in 3.7% paraformaldehyde, 0.1% glutaraldehyde and permeabilized in 0.15 mg ml −1 saponin in dPBS. Cells were incubated with annexin A2 antibody (4 μg ml −1 , clone A-15, Santa Cruz) and LAMP1 (5 μg ml −1 , clone NB120, Novus Biologicals) for 90 min. Annexin A2–GFP transfectants were incubated with only the LAMP1 primary antibody. Donkey anti-rabbit IgG-Alexa Fluor 488 conjugated (5 μg ml −1 ) and rabbit anti goat IgG Alexa Fluor 633-conjugated (5 μg ml −1 ) were used as secondary antibodies (Molecular Probes). Cells were visualized using an Olympus IX70 inverted microscope equipped with an I.P. Lab Spectrum imaging software (Scanalytics Inc. Fairfax, VA). For time-lapse fluorescence Annexin A2–GFP DCs were incubated with LysoTracker for 30 min and either left untreated or exposed to WD. Cells were imaged every 20 min for 3 h. At least 40 cells were analysed per each experimental condition. Images were processed as described above [40] . Preparation of liposomes and annexin A2 Binding Dioleoyl-sn-glycero-3-phospho-l-serine (DOPS), 2-dioleoyl-sn-glycero-phosphocholine (DOPC) and cholesterol were purchased from Avanti Polar Lipids (Alabaster, AL). Lipids were dissolved in chloroform and lyophilized by solvent removal with a rotary evaporator and vacuum oven overnight. The lipid film was hydrated in 0.9% saline and unilamellar liposomes obtained by sonication and extrusion through polycarbonate membrane with a pore size of 0.05 μm. Liposomes were gassed with a stream of Argon gas and stored at 4 °C overnight, until the start of the binding studies. Liposomes (10 μl) were spotted on formvar-coated stained with 1% phosphotungstic acid and viewed with a Jeol JEM-1200EX transmission electron microscope at 80 kV. In some experiments, recombinant annexin A2 (5 μg) was incubated with DOPS/Cholesterol, DOPS, and DOPC liposomes for 30 min at 37 °C in 150 mM NaCl, ±0.4 mM Ca ++ , pH 7.15 and 7.4. Binding was analysed via western blotting following the separation of liposome-bound and unbound annexin A2 by ultracentrifugation at 35,000 r.p.m. for 1 h at 4 °C. FACS analysis of endosomal liposomal-annexin A2 binding 50 μg of control and WD-treated endosomes were incubated with fluorescently labelled (Sigma MINI67) DOPS/cholesterol and DOPS liposomes in 150 mM NaCl pH 7.4, in presence or absence of 0.4 mM Ca 2+ and recombinant annexin A2 (5 μg) at 37 °C for 1 h. Endosomes were analysed by FACS using a flow cytometer LSR II (Becton Dickinson). ELISA IL-1β production from control and treated primary dendritic cells was quantified using an OptEIA ELISA kit (BD Pharmingen). Calcium assay and pH measurement Calcium concentrations were measured using the QuantiChrom calcium assay kit (BioAssay Systems, Hayward, CA, USA). Cytosolic pH measurements were performed by labelling 10 μg of cytosolic fractions with 1.5 μl of Lysosensor Green (Invitrogen). Fluorescence emission scans were collected on a spectrofluorimeter between 460–600 nm (excitation wavelength). Ellipsometry studies Silicon slides [41] were flushed with deionized water and dipped into 0.01 mol l −1 . HEPES, 0.14 mol l −1 NaCl, 0.1% BSA, and 5 mmol l −1 CaCl 2 (HBSA, pH 7.5). Phospholipid bilayers (50 μM) comprised (DOPS)/cholesterol (1:1), DOPS, or DOPC were formed on the reflective silicon slides [42] . The bound bilayers were transferred to an ellipsometry cuvette containing 1 ml of stirring HBSA. To study the effects of pH and/or calcium on annexin A2 binding to phospholipid bilayers, HBSA was replaced with buffers consisted of 150 mM NaCl of varying pH with the presence or absence of calcium. Recombinant annexin A2 (5 μg ml −1 ) was added for each condition, and binding was monitored with a thin film ellipsometer (Rudolph & Sons, Fairfield, NJ, USA). 2D-DIGE protein expression profiling of cytosolic fractions A weight of 25 μg of cytosolic proteins from WD-treated or untreated cells were labelled with 400 pmol of either Cy3 (green) or Cy5 (red) for 30 min on ice. The labelling reaction was stopped with 10 mM lysine. Cy3- and Cy5-labelled proteins were mixed in 7 M urea, 2 M thiourea, 4% CHAPS, 40 mM dithiothreitol, 1% IPG buffer (pH 4–7), 0.002% bromophenol blue and applied to Immobiline DryStrips (24 cm, pH 4–7; GE Healthcare). Isoelectric focusing was performed with an Ettan IPGphor II apparatus (GE Healthcare). After isoelectric focusing, the proteins were reduced and alkylated by successive 15-min treatments with equilibration buffer containing 2% dithiothreitol followed by 2.5% iodoacetamide. The proteins were then resolved in 4–20% SDS–PAGE gels, using an Ettan DALTsix instrument (GE Healthcare). Gel images were acquired on a Typhoon 9400 scanner (GE Healthcare) and analysed using DeCyder Software (V6.0, GE Healthcare). LTQ-tandem MS/MS sequencing In situ trypsin digestion of protein fragments was performed after reductive alkylation using 25 ng μl −1 of trypsin in 50 mM ammonium bicarbonate buffer, at pH 8.9. for 45 min. The trypsin digestion was stopped with trifluoroacetic acid to a final concentration of 0.1%. The samples were desalted for MS/MS analysis using the ZipTip on C18 (Millipore). LTQ-MS/MS sequencing of tryptic peptides from individual 2D-spots was performed using nanospray LC-MS/MS on a LTQ linear ion trap mass spectrometer (LTQ, Thermo, San Jose, CA, USA) interfaced with a TriVersa NanoMate nanoelectrospray ion source (Advion BioSciences, Ithaca, NY, USA). The sequences of each peptide were determined using the LTQ software analysis MS database searching with MASCOT algorithm (from Matrix Science). Statistical analysis All data are reported as mean±s.e.m. Statistical significance of the difference between experimental groups in cases of multiple means comparisons was determined by one-way analysis of variance (ANOVA) followed by the Tukey post hoc analysis using GraphPad Prism version 5 (Graph-Pad Software, Inc.). How to cite this article: Scharf, B. et al . Annexin A2 binds to endosomes following organelle destabilization by particulate wear debris. Nat. Commun. 3:755 doi: 10.1038/ncomms1754 (2012).